An artificial PPR scaffold for programmable RNA recognition Pentatricopeptide repeat (PPR) proteins control diverse aspects of RNA metabolism in eukaryotic cells. Although recent computational and structural studies have provided insights into RNA recognition by PPR proteins, their highly insoluble nature and inconsistencies between predicted and observed modes of RNA binding have restricted our understanding of their biological functions and their use as tools. Here we use a consensus design strategy to create artificial PPR domains that are structurally robust and can be programmed for sequence-specific RNA binding. The atomic structures of these artificial PPR domains elucidate the structural basis for their stability and modelling of RNA–protein interactions provides mechanistic insights into the importance of RNA-binding residues and suggests modes of PPR-RNA association. The modular mode of RNA binding by PPR proteins holds great promise for the engineering of new tools to target RNA and to understand the mechanisms of gene regulation by natural PPR proteins. RNA plays many essential roles in cells, from information transfer and regulation of gene expression to the scaffolding of macromolecular structures and catalysis. Indeed the chemical and structural flexibility of RNA likely enabled self-replicating RNAs to kick start life itself, predating the first proteins [1] . Nevertheless, in modern biological systems proteins and RNAs are intimately linked and depend on each other for their functions in cells. Physical binding of proteins to RNA controls every aspect of an RNA’s life, from transcription to decay [2] . The ability to manipulate the properties of RNA using engineered RNA-binding proteins is an attractive prospect for biotechnological and therapeutic applications. Furthermore, the need for new methods to determine the functions of RNAs has become even more critical given the unprecedented complexity of cellular transcriptomes that has recently been revealed using massively parallel sequencing [3] , [4] , [5] . Although robust technologies have now emerged that enable the site-specific manipulation of DNA in living cells [6] , equivalent technologies for the manipulation of RNA are still in their infancy [7] . Computational studies of a large family of RNA-binding proteins, known as pentatricopeptide repeat (PPR) proteins, have predicted that they bind their targets in a modular and sequence-specific manner [8] , [9] , [10] . PPR proteins contain a repeated motif that is typically 35 amino acids in length and folds into two anti-parallel alpha helices [11] , [12] , [13] , [14] . Natural proteins have been observed to contain between two and thirty individual PPRs [15] . Some PPR proteins appear to consist almost entirely of tandem PPRs, while some contain other domains, such as endonuclease or protein interaction domains [15] , [16] , [17] . Statistical correlations between specific PPR residues and RNA bases within their binding sites have elucidated a potential code for RNA recognition by PPR proteins [8] , [9] , [10] . A significant correlation was found between the identities of amino acids at positions 4 and 34 and particular bases within the RNA footprint [8] , [9] , [10] . Furthermore, one study indicated that the identity of the amino acid at position 1 might fine-tune base recognition [9] . Recently the structures of two distinct PPR-RNA complexes have been described at atomic resolution [18] , [19] . Surprisingly, although some elements of a modular recognition code were observed, the majority of the RNA chains in both of these structures were bound independently of the sequence of their RNA bases. A key limitation in studying and engineering PPR proteins is their highly insoluble nature when expressed in heterologous systems. For example, extensive mutagenesis and truncations of the PPR10 protein were required for production of soluble protein for crystallization studies [18] . This problem has severely delayed the elucidation of the mechanisms of PPR-RNA binding and their potential use as tools. To understand the modes by which PPR proteins bind RNA better, and to develop PPR scaffolds that would enable robust and reliable recognition of RNA targets of interest, we designed synthetic PPR domains based on the conservation of residues within PPRs throughout evolution. These synthetic PPR domains are highly soluble and, via an appropriate choice of amino acids at position 4 and 34, we can make them bind RNA in a predictable, sequence-specific manner. Structural analysis of these proteins reveals the mechanistic details of how interactions between and within individual PPR modules stabilize the elongated array. Furthermore, we suggest that the overall shape of the PPR scaffold is partially dependent on the amino acids that mediate RNA association. This engineered PPR scaffold enables the predictable binding of RNA targets and provides a starting point to use engineered PPR proteins to rationally manipulate cellular gene expression. By comparing our atomic models with the solved PPR structures, we could propose several models describing the interaction of the targeted nucleotides with the individual cPPR motifs. The canonical mode of RNA binding by PPR proteins can now be unambiguously redesigned for technological applications as demonstrated by the present biochemical and structural studies. A consensus PPR protein scaffold To bypass the problems associated with the extreme insolubility of natural PPR proteins, we pursued a consensus design strategy. This approach uses large multiple sequence alignments of related protein sequences to determine the most over represented amino acids at each position within a domain [20] , [21] , [22] , [23] . Because of their enrichment over vast evolutionary timescales, these amino acids are predicted to be best suited to enhance that domain’s activity or stability. This approach has been very successful in designing protein-binding repeat proteins with massively enhanced solubility and stability [21] , [24] , [25] but had not been applied to RNA-binding proteins. A particular advantage for PPR proteins is that there are many of these proteins in each eukaryotic genome, for example, there are seven in humans and over 400 in most higher plants, and each protein contains multiple PPRs, between 2 and 30 per protein. This provides a rich resource of sequence data from which to draw a consensus. We collected and curated a set of 23,916 PPR sequences obtained from the UniProtKB database. The consensus of over represented amino acids revealed a strong enrichment for particular amino acids at each position ( Fig. 1a ). We used this consensus as the basis for a synthetic consensus PPR protein (‘cPPR’) ( Fig. 1b ). We used the most enriched amino acid at each position, with the exception of position 11, where cysteine was replaced with glycine to exclude the possibility of undesirable disufide bonds that may interfere with folding. The design of the final cPPR protein consisted of eight identical repeats because (i) it is of a manageable size for cloning and expression, (ii) based on previous experience working with pumilio and FBF homology (PUF) proteins this likely strikes a balance between effective binding and non-specific association [26] and (iii) it would be predicted to be able to bind a contiguous RNA [8] . In addition to the repeated consensus units, two extra features were added to the cPPR design: nucleating N-terminal cap residues (Met-Gly-Asn-Ser) and a C-terminal solvating helix. The Met-Gly-Asn-Ser N-terminal cap was used because statistically Gly, Asn and Ser have the highest propensities to occur at these N-terminal positions in α helices [27] . The C-terminal solvating helix was added after the final consensus repeat to prevent unfolding, according to the successful consensus tetratricopeptide repeat domain design of ref. 28 . Overexpression of the cPPR protein in Esherichia coli revealed that, unlike natural PPR proteins, the majority of the protein was found in the soluble fraction after cell disruption ( Supplementary Fig. 1 ). We used thermal denaturation to examine the stability of our cPPR in comparison with the best-characterized naturally occurring PPR protein, PPR10 from maize. We show that the Tm value of the PPR10 protein is 39 °C while the Tm value for our designed PPR protein is 55 °C, confirming the markedly improved stability of the cPPR scaffold ( Supplementary Fig. 2 ). 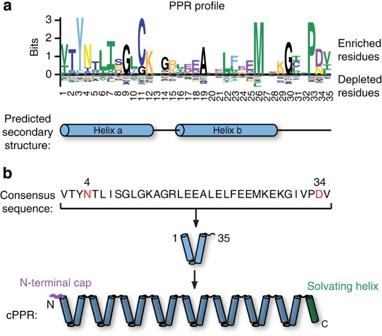Figure 1: Design of a consensus PPR protein scaffold. (a) A sequence logo derived from all identified PPRs in the UniProtKB database and its predicted secondary structure. Amino acids are colour coded according to the physiochemical properties of their side chains: small (A, G) in black, nucleophilic (C, S, T) in blue, hydrophobic (I, L, V, M, P) in green, aromatic (F, W, Y) in red, acidic (D, E) in purple, amides (Q, N) in yellow and basic (H, K, R) in orange. Amino acids are numbered based on the Pfam model for PPR, which functions as a minimal unit29. Residue 34 is also defined as ‘ii’ according to ref.29, while the numbering scheme used by ref.61is shifted to the N terminus by two amino acids such that amino acids 1, 4 and 34 in the Pfam model are annotated as 3, 6 and 1, respectively. (b) The PPR consensus sequence and its assembly into an eight-repeat protein flanked by stabilizing elements. Figure 1: Design of a consensus PPR protein scaffold. ( a ) A sequence logo derived from all identified PPRs in the UniProtKB database and its predicted secondary structure. Amino acids are colour coded according to the physiochemical properties of their side chains: small (A, G) in black, nucleophilic (C, S, T) in blue, hydrophobic (I, L, V, M, P) in green, aromatic (F, W, Y) in red, acidic (D, E) in purple, amides (Q, N) in yellow and basic (H, K, R) in orange. Amino acids are numbered based on the Pfam model for PPR, which functions as a minimal unit [29] . Residue 34 is also defined as ‘ii’ according to ref. 29 , while the numbering scheme used by ref. 61 is shifted to the N terminus by two amino acids such that amino acids 1, 4 and 34 in the Pfam model are annotated as 3, 6 and 1, respectively. ( b ) The PPR consensus sequence and its assembly into an eight-repeat protein flanked by stabilizing elements. Full size image Modular RNA binding by engineered cPPR domains We hypothesized that because all eight synthetic PPR repeats within the cPPR were identical, if each repeat bound a specific RNA base, then the cPPR might bind specifically a particular RNA homopolymer. The particular amino acids found at positions 4 and 34 of our cPPR are asparagine and glutamate, respectively (‘ND’). Bioinformatic and recent structural analysis predicted that this combination would bind uracil [8] , [9] , [10] . We performed RNA electrophoretic shift assays with RNA homopolymers and observed specific binding of our designed cPPR to poly(U) RNA but no other RNA homopolymer ( Fig. 2 ). Thus, we confirmed in our experiments that our designed protein binds RNA according to the ‘PPR code’. This also suggests that the majority of the nucleotidic sequences targeted by PPR proteins are likely to correspond to uracil-rich sequences. 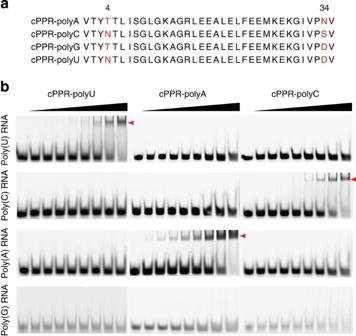Figure 2: RNA-binding preferences of consensus PPR proteins. (a) Sequences of the cPPR repeats with the nucleotide binding residues indicated in red. (b) Purified proteins were titrated against homopolymeric RNA probes in an RNA electrophoretic mobility shift assay (EMSA). Complexes formed between predicted cognate RNA-protein pairs are indicated with red arrows and demonstrate that high specificity of each cPPR protein for its cognate RNA target. Figure 2: RNA-binding preferences of consensus PPR proteins. ( a ) Sequences of the cPPR repeats with the nucleotide binding residues indicated in red. ( b ) Purified proteins were titrated against homopolymeric RNA probes in an RNA electrophoretic mobility shift assay (EMSA). Complexes formed between predicted cognate RNA-protein pairs are indicated with red arrows and demonstrate that high specificity of each cPPR protein for its cognate RNA target. Full size image Mutating the amino acids at positions 4 and 34 to the other most common pairs of residues enabled us to confirm predictions that threonine at position 4 and asparagine at position 34 (‘TN’) bound adenine, and that asparagine at position 4 and serine at position 34 (‘NS’) bound cytosine ( Fig. 2 ). Elucidation of the amino acid code for recognition of guanine proved challenging because the propensity of G tracts to form stable quadruplex structures [29] might mask any potential cPPR binding. To overcome this obstacle we designed a cPPR variant that bound a heteropolymeric RNA target containing a single guanine, the nanos-response element (NRE). The designed cPPR had positions 4 and 34 of each repeat modified so that it would bind the NRE sequence (cPPR-NRE, Fig. 3a ). The cPPR-NRE bound tightly to the NRE in contrast to the NRE RNA with a G2C mutation ( Fig. 3b , Supplementary Table 1 ) or G2A and G2U mutations ( Supplementary Fig. 3 ), confirming that the T4D34 combination we had incorporated in the cPPR-NRE based on bioinformatic predictions bound guanine specifically. Incorporation of the N4S34 combination, found to bind cytosine, in place of T4D34 created a cPPR that bound the G2C mutant NRE sequence with similar affinity to the original cPPR-NRE:NRE RNA complex. 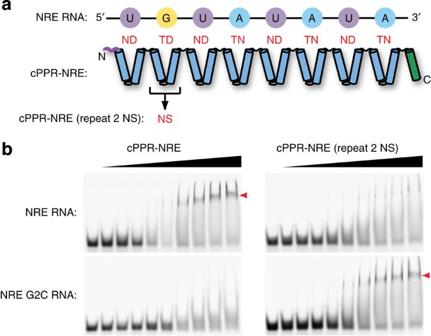Figure 3: Programmable RNA binding by engineered consensus PPR proteins. (a) Schematic view of the cPPR protein designed to bind the nanos response element (NRE, 5′-UGUAUAUA-3′). cPPR-NRE(repeat 2 NS) carries a mutated repeat in position 2. (b) EMSA demonstrates that cPPR-NRE recognizes the NRE element more efficiently than the NRE sequence carrying a G-to-C mutation at position 2 (NREG2C, 5′-UCUAUAUA-3′). The cPPR-NRE (repeat 2 NS) mutant protein binds the mutated NREG2C probe more tightly, as predicted from the code determined from homopolymer assays. This confirmed the specificity of the TD amino-acid combination for guanine. Complexes formed between predicted cognate RNA–protein pairs are indicated with red arrows. Figure 3: Programmable RNA binding by engineered consensus PPR proteins. ( a ) Schematic view of the cPPR protein designed to bind the nanos response element (NRE, 5′-UGUAUAUA-3′). cPPR-NRE(repeat 2 NS) carries a mutated repeat in position 2. ( b ) EMSA demonstrates that cPPR-NRE recognizes the NRE element more efficiently than the NRE sequence carrying a G-to-C mutation at position 2 (NREG2C, 5′-U C UAUAUA-3′). The cPPR-NRE (repeat 2 NS) mutant protein binds the mutated NREG2C probe more tightly, as predicted from the code determined from homopolymer assays. This confirmed the specificity of the TD amino-acid combination for guanine. Complexes formed between predicted cognate RNA–protein pairs are indicated with red arrows. Full size image To further explore the potential of cPPRs to predictably target RNAs, we designed a cPPR that specifically bound the RNA recognition sequence of the human MBNL1 protein [30] ( Supplementary Fig. 4a,b ). In addition, we show that further alteration of this cPPR, by introducing two point mutations predicted to change the nucleotide recognition properties, enables the specific recognition of an RNA almost entirely composed of G and C nucleotides ( Supplementary Fig. 4b ), further demonstrating the specificity of RNA recognition by cPPRs. To examine the roles of individual repeats within the cPPR in RNA binding we produced cPPRs of various lengths, with 1, 2, 3, 4, 5, 6 or 7 repeats, in addition to the original 8 repeat cPPR-NRE. We show that these proteins can be expressed and purified in increasing amounts with the 8-repeat protein performing best ( Supplementary Fig. 5 ). Furthermore, we show that only cPPRs with 6, 7 and 8 repeats bind RNA significantly and that the affinity increases with repeat number. In addition, binding of the cPPR-polyA protein to an adenine homopolymer with a single cytosine at the centre was reduced compared with poly(A) RNA ( Supplementary Fig. 6 ). All together, the presented data demonstrate that repeats 2, 3, 4 and 5 from our cPPR recognize individual nucleotides and strongly suggest that all repeats within the cPPR are contributing to RNA recognition. These results biochemically validate the computationally predicted code for base recognition as well as previous structural observations [18] , and demonstrate that our engineered cPPRs can bind RNAs in a programmable manner. Crystal structures of cPPR proteins We then tried to obtain structural information on five cPPR proteins, specifically designed to bind to poly(A), poly(U), poly(C), poly(G) and NRE RNA sequences, to further understand the PPR scaffold’s stability and RNA association. Although these proteins are highly similar at the primary sequence, their crystallographic behaviour was significantly different. Four of these proteins crystallized (cPPR-polyA, cPPR-polyC, cPPR-polyG and cPPR-NRE) and gave reproducible and diffracting crystals. Moreover, we obtained various crystal forms of cPPR-polyC and cPPR-NRE. After diffraction data analyses, these proteins appeared to have crystallized in various space groups with different unit cell parameters, while cPPR-polyG crystallized in a unique space group (data not shown). We also observed a large variety of diffraction limits for these protein crystals ranging from 2.0 to 3.8 Å ( Table 1 , with sample electron densities in Supplementary Fig. 7 ). Atomic structures had to be solved using anomalous data measured from a selenomethionine-derivatized protein crystal of cPPR-NRE ( Fig. 4a ) as the strategy of using the already available atomic models to perform tri-dimensional searches was to be unsuccessful. This failure to solve our crystal structures using molecular replacement indicated that the cPPRs adopted an overall fold that was different from the known examples of PPR structures. The cPPR-polyA, cPPR-polyC and cPPR-polyG structures were then solved by molecular replacement using the cPPR-NRE model ( Fig. 4a and Supplementary Fig. 7 ). The overall cPPR protein structures are repetitions of pair of helices packing against each other. Structural comparisons with previously solved PPR motifs present in mtRNAP, PPR10, PRORP1 and THA8 showed strong conservation of the individual PPR unit ( Supplementary Fig. 8 ), confirming that our engineered PPR motifs fold like the natural ones ( Fig. 4a ). Interestingly only five repeats for cPPR-NRE and six repeats for cPPR-polyG and cPPR-polyA could be built, respectively, while the entire protein chain was clearly visible for cPPR-polyC ( Fig. 4a and Supplementary Fig. 7e ). Analysis of the protein crystal content showed that proteins were not degraded during crystallization ( Supplementary Fig. 9a–c ). Furthermore, limited proteolysis with the protease subtilisin revealed no significant differences in the protease susceptibility between different cPPR proteins ( Supplementary Fig. 9d ). Therefore, the absence of individual PPR motifs within the NRE-, poly(A)- and poly(G)-binding cPPR atomic models was most likely a result of these proteins’ behaviour in the crystallization process, revealing the inherent flexibility of the PPR scaffold. Moreover, it potentially indicates that the residues involved in RNA binding affect the overall topology of the PPR scaffold. Table 1 Data collection and refinement statistics. 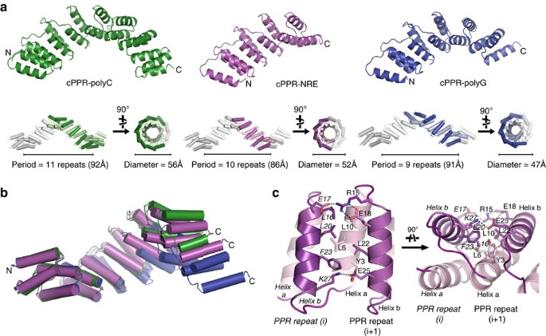Figure 4: Atomic structures of consensus PPR proteins. (a) Overall view of the atomic models for cPPR-polyC, cPPR-NRE and cPPR-polyG. The proteins form superhelices with the indicated period length and diameter values. The cPPR-polyA atomic structure has an identical period length and diameter value as cPPR-polyG (Supplementary Fig. 7eandTable 1); therefore, it was not included for clarity. Proteins are coloured in green, purple and blue for cPPR-polyC, cPPR-NRE and cPPR-polyG, respectively. Symmetry related molecules from the crystal lattice are coloured in light grey. The parameters of the superhelix are indicated. (b) Superposition of the three cPPR structures shows the amplification of the small difference existing between the interactions of our engineered PPR modules. (c) The observed helical shift results from a slight variation in the packing of helix b against helix a between individual PPR repeats. Protein is shown as a cartoon and cPPR-NRE is shown as example. Contacts between adjacent PPR motifs are mediated by various hydrophobic residues and several salt bridges. Residues are labelled and coloured according to atom type (carbon: purple, oxygen: red, nitrogen: blue). Hydrogen bonds are indicated by dash lines. Full size table Figure 4: Atomic structures of consensus PPR proteins. ( a ) Overall view of the atomic models for cPPR-polyC, cPPR-NRE and cPPR-polyG. The proteins form superhelices with the indicated period length and diameter values. The cPPR-polyA atomic structure has an identical period length and diameter value as cPPR-polyG ( Supplementary Fig. 7e and Table 1 ); therefore, it was not included for clarity. Proteins are coloured in green, purple and blue for cPPR-polyC, cPPR-NRE and cPPR-polyG, respectively. Symmetry related molecules from the crystal lattice are coloured in light grey. The parameters of the superhelix are indicated. ( b ) Superposition of the three cPPR structures shows the amplification of the small difference existing between the interactions of our engineered PPR modules. ( c ) The observed helical shift results from a slight variation in the packing of helix b against helix a between individual PPR repeats. Protein is shown as a cartoon and cPPR-NRE is shown as example. Contacts between adjacent PPR motifs are mediated by various hydrophobic residues and several salt bridges. Residues are labelled and coloured according to atom type (carbon: purple, oxygen: red, nitrogen: blue). Hydrogen bonds are indicated by dash lines. Full size image The four structures, despite being quite similar with each other due to their very similar amino acid sequence, do have noticeable variations, in particular in the observed curvature of the right-handed helix formed by the individual PPR motifs ( Fig. 4b ). The array of tandem PPR motifs stack on each other to produce a superhelix with a variable curvature that induces different helical periods ranging from 86 Å for cPPR-NRE to 91–92 Å for cPPR-polyA, cPPR-polyG and cPPR-polyC ( Fig. 4a,b ). The helix diameters are markedly different ranging from 47 Å for cPPR-polyA and cPPR-polyG to 56 Å for cPPR-polyC, with an intermediate value of 52 Å for cPPR-NRE. Consequently the superhelix period contains 9 (cPPR-polyA and cPPR-polyG), 10 (cPPR-NRE) and 11 (cPPR-polyC) PPR repeats, coincident with the increase in the superhelix diameter ( Fig. 4a,b ). As the number of PPR repeats contained in one complete turn of the superhelix is increasing, the packing angles between individual PPR motifs are reduced from 40 to 36 and 33 degrees for cPPR-polyA/cPPR-polyG, cPPR-NRE and cPPR-polyC, respectively. The reduction of the angle is likely caused by a slight variation in the packing of the helix b against helix a within and between individual PPR motifs ( Fig. 4b,c ). Contacts between adjacent PPR motifs are mediated by various hydrophobic residues. Residues L16, L20 and F23 from helix b of one PPR motif form hydrophobic interactions with residues Y3, L6, L10 from helix a and L22 from helix b of the following PPR motif ( Fig. 4c ). Together with this hydrophobic core, salt bridges between, on the one hand residue E17 (helix b of PPR motif 1) and residues R15, E18 (helix b of PPR motif 2), and, on the other hand residue K27 (helix b of PPR motif 1) and E25 (helix b of PPR motif 2), fine-tune the strength of association and the orientation of each PPR motif with respect to the next one ( Fig. 4c ). The residues mediating the packing between the two helices composing each PPR motif are identical in the four crystallized proteins. Thus, the observed variations in curvature highlight the capacity of individual PPR repeats to pack variably against each other and indicate that the RNA-binding residues at positions 4 and 34 might influence the overall architecture of PPR arrays, most likely through a slight change in the electrostatic properties. This flexibility could also reflect a pre-requisite to accommodate RNAs of various sequences, in particular if they contain purines rather than pyrimidines as these would require pockets that allow deeper insertion. Accordingly, we observe a larger angle between neighbouring PPR motifs in cPPR-polyG and cPPR-polyA than in cPPR-polyC ( Fig. 4a,b ). cPPR-RNA models A previous study of PPR10 observed direct hydrogen bonding of adenine, guanine and uracil by S, T and N residues, respectively, at position 4 of the corresponding PPR modules [18] . Specific recognition of cytosine has not previously been observed, although direct hydrogen bonding by N4 was predicted [18] . In our structures, the electrostatic properties highlight the proposed nucleic acid binding groove in the inner face of the superhelix ( Fig. 5a ). The three residue loops (aa 13–15) linking helix a to helix b within each PPR motif, line up at the opposite side from the putative base binding sites in our cPPR structures. Located at the extremity of this short loop, the lysine residue at position 12 has a positive charge that could stabilize a negatively charged phosphate group ( Fig. 5a ). We modelled the interaction between a particular nucleotide type and the corresponding cPPR repeat using PPR10/PSAJ RNA structure as a guide ( Supplementary Fig. 10 ). The four types of bases (cytosine, guanine, uracil and adenine) for which we obtained atomic models of the cognate cPPR can be positioned individually at hydrogen bonding distances from the amino-acid side chains at position 4 and 34 ( Fig. 5b–d ). Because the recognition of cytosine by a PPR repeat was not observed in the PPR10-PSAJ RNA structure [18] , or any other structure to date, we modelled cytosine recognition based on uridine. Despite the absence of direct hydrogen bonds between the hydroxyl group and the D34 position of PPR10 or our cPPR, uridine is recognized specifically. We speculate that hydration, tautomeric equilibrium or overall charge are factors that likely play a critical role in the stabilization of cytosine versus uridine by individual PPR motifs. 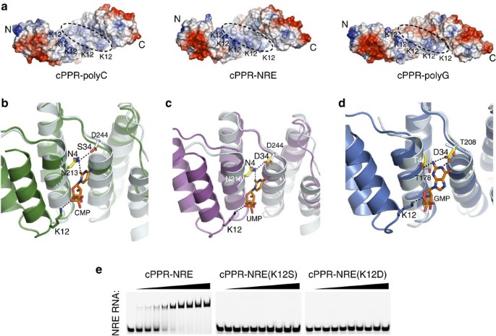Figure 5: RNA-binding residues of consensus PPR proteins. (a) The electrostatic properties highlight the nucleic acid binding groove on the inner face of the superhelix. The locations of the residues at positions 4 and 34 in cPPR-polyC and cPPR-polyG are indicated by dashed ellipses. The three types of nucleobase (C, U and G) for which we designed a corresponding repeat can be positioned individually at hydrogen bonding distances from the amino-acid side chains at position 4 and 34 of the cPPR sequences found in cPPR-polyC (b), cPPR-NRE (c) and cPPR-polyG proteins (d). Each cPPR is superimposed onto the atomic model of PPR10 as shown inSupplementary Fig. 10(PDB 4M59). The PPR10 protein is shown as cartoon and colored in light grey. Residues involved in RNA binding and individual nucleotides are shown as sticks and coloured according to atom type (carbon: yellow or orange, oxygen: red, nitrogen: blue). Large letter labels refer to residue numbers in the cPPR, small letter labels refer to the residue numbering in the PPR10 sequence. Potential hydrogen bonds between the modelled nucleotide and the cPPR side chain atoms are shown as dashed lines. (e) Mutation of the lysine at position 12 of each repeat to either serine (K12S) or aspartate (K12D) abolishes the binding of these proteins to RNA. Figure 5: RNA-binding residues of consensus PPR proteins. ( a ) The electrostatic properties highlight the nucleic acid binding groove on the inner face of the superhelix. The locations of the residues at positions 4 and 34 in cPPR-polyC and cPPR-polyG are indicated by dashed ellipses. The three types of nucleobase (C, U and G) for which we designed a corresponding repeat can be positioned individually at hydrogen bonding distances from the amino-acid side chains at position 4 and 34 of the cPPR sequences found in cPPR-polyC ( b ), cPPR-NRE ( c ) and cPPR-polyG proteins ( d ). Each cPPR is superimposed onto the atomic model of PPR10 as shown in Supplementary Fig. 10 (PDB 4M59). The PPR10 protein is shown as cartoon and colored in light grey. Residues involved in RNA binding and individual nucleotides are shown as sticks and coloured according to atom type (carbon: yellow or orange, oxygen: red, nitrogen: blue). Large letter labels refer to residue numbers in the cPPR, small letter labels refer to the residue numbering in the PPR10 sequence. Potential hydrogen bonds between the modelled nucleotide and the cPPR side chain atoms are shown as dashed lines. ( e ) Mutation of the lysine at position 12 of each repeat to either serine (K12S) or aspartate (K12D) abolishes the binding of these proteins to RNA. Full size image Interestingly, the phosphate group of our modelled nucleotide is at hydrogen bonding distance from the above mentioned lysine 12 residues, suggesting that they play an important role in stabilizing the phosphate backbone of the targeted nucleic acid sequence ( Fig. 5b–d ). We generated cPPR-NRE mutants where the lysines at position 12 of each repeat were mutated to either serine or aspartate. We found that, although these mutated proteins express as well as the parental protein, their capacity to bind RNA is completely abolished ( Fig. 5e ), confirming our prediction that K12 plays a key role in stabilizing bound RNA. One important aspect of our nucleic acid docking resides in our inability to model more than two consecutive nucleotides. Indeed, the average distance between each nucleotide binding pocket in the PPR motif is between 8.5 and 10.5 Å ( Supplementary Table 2 ). Such spacing is larger than the typical distance separating two consecutive nucleotides, even if their sugar ring adopts a C2′-endo conformation. We hypothesized that a conformational change would be required to bind the octanucleotide RNA targets. The ability of repeat proteins to undergo substantial conformational changes upon ligand binding has been well characterized for TALE proteins, which compact significantly on DNA binding [31] , [32] , [33] . The protein importin β is another example of repeat-containing proteins, which undergoes a significant compaction upon cargo binding. Although less well studied for PPR proteins, the natural PPR protein PPR10 adopts a more compact fold upon association with RNA [8] , [18] , and this property is likely conserved in our engineered proteins. In summary, we used protein engineering to build stable and soluble PPR proteins with predefined RNA targets. The consensus design strategy results in an artificial protein that is the statistical average of all known PPR proteins, without having high identity to any one natural protein ( Supplementary Table 3 ). Our structures of the designed cPPR proteins provide clues as to why natural PPR proteins may have limited solubility. We observed that, compared with natural PPR proteins, hydrophobic interactions organizing the overall PPR scaffold are shielded from the solvent by salt bridges between residues at position 17, 27 and 15, 18, 25. This is reminiscent of the binding between NSUN4 and MTERF1 proteins, where salt bridges also flank hydrophobic interactions to provide a very stable interaction interface [34] . In addition, consensus design enabled core structural characteristics of PPRs to be elucidated without interference from the idiosyncratic features present in individual natural proteins. Our strategy revealed a number of features that may facilitate rational engineering to improve protein properties in the absence of large numbers of homologous sequences. We observed that the interactions between each cPPR repeat give rise to some flexibility within each designed PPR scaffold, as exemplified by the variation of helical period. Such plasticity may modulate their RNA binding properties, particularly in their capacity to accommodate the larger purine nucleobases. The stability and robust RNA-binding properties of our designed PPR proteins could be used to further examine the contributions of different residues within natural PPRs to protein folding and RNA-binding by transplanting them into the cPPR scaffold. Interestingly, in the bioinformatic studies of ref. 9 a correlation between the amino acid at position 1 of the PPR and the predicted nucleotide specificity was detected, although this was less important than the identity of the residues at positions 4 and 34. In this model the presence of phenylalanine at position 1 can sometimes alter the predicted binding specificity, for example with asparagine at both positions 4 and 34 binding to adenine and guanine is favoured, while binding to adenine and cytosine is predicted to be preferred if valine is found at position 1. Altering the amino acid at position 1 could generate further cPPR variants with altered affinities or degenerate nucleotide recognition properties. Such properties could be critical if these proteins would be used as carriers for non-natural nucleic acids such as locked nucleic acids or unnatural base pairs. The modular mode of DNA binding by TALE proteins has opened up the possibilities of using designed DNA-binding proteins for many applications. The very high levels of sequence similarity between repeats enable the binding preferences of TALEs to be modified with very few context-dependent variations in affinity or specificity. This is not true, however, for the only other well-characterized RNA-binding repeat proteins of the pumilio and FBF homology (PUF) family. Although biochemical and structural studies of PUFs have shown that they interact with RNA in a modular manner, their diverse repeats make designing RNA-binding proteins free from context-dependent effects or with predictable binding affinities challenging. Furthermore, the structures of PUF proteins provide certain key limitations to their possible applications; their overall fold limits the number of repeats that can be assembled contiguously and the tendency for some bases of the target RNA to flip out from the RNA-binding surface can result in reduced RNA-binding specificity [35] , [36] , [37] , [38] . PPR proteins have a number of desirable features that make the development of their applications in biotechnology and synthetic biology quite appealing, now that a robust soluble and fully synthetic PPR module has been developed. We showed that our individual PPR modules can be combined within the engineered cPPR proteins with the capacity to modify their binding specificities to single-nucleotide level, providing further evidence of their modularity. We thus demonstrate that they might be engineered to target and manipulate RNAs of interest, as has been the case for PUFs [7] , [26] , [37] , [39] , [40] , [41] , [42] , [43] , [44] , [45] , [46] . Here we focused on engineered proteins with eight PPRs. Many naturally occurring RNA-binding proteins specifically recognize eight nucleotides; however, this is sufficient for them to selectively regulate specific developmental processes, although they often do so by binding multiple different RNAs [47] . It should be noted that miRNAs often recognize their target mRNAs using as few as 6–8 nucleotides (the seed region) at their 5′ end, with relatively little contribution from the remaining miRNA [48] . However, we recognize that for many applications in biotechnology and synthetic biology it would be desirable to be able to target only one species of RNA within the entire transcriptome. Natural PPR proteins have been observed to contain between two and thirty individual PPRs [15] , providing considerable flexibility in the complexity of the RNA sequences they might bind, and many opportunities to balance specificity and affinity. Moreover, the PPR proteins characterized to date operate in mitochondria, chloroplasts and nuclei, locations where the most common RNA-directed tool, RNA interference, cannot function or functions poorly to target RNAs [48] , [49] . As proteins that contain PPRs have often been observed to contain many other domains with diverse roles in RNA metabolism, such as RNA cleavage, modification and control of translation [15] , these proteins are de facto structurally compatible for fusion with partner proteins. These qualities will likely be very useful for making new research tools to manipulate aspects of RNA biology that have been neglected due to a lack of appropriate reagents and for controlling gene networks to build cells with new properties in synthetic biology. Design and synthesis of consensus PPR (cPPR) sequences PPR sequences obtained using PSI-BLAST from the UniProtKB database [50] . Multiple identical sequences were removed and sequences were aligned using ClustalW [51] . The aligned sequences were used to generate a Position-Specific Scoring Matrix using BLAST [52] , and this was used to derive a consensus sequence using Seq2Logo 2.0 (ref. 53 ). The cPPR coding sequence was designed based on eight tandem repeats with the most enriched amino acid at each position, with the exception of position 11, where Cys was replaced with Gly. N-terminal cap residues (Met-Gly-Asn-Ser) and a C-terminal solvating helix were added to the final design (Val-Thr-Tyr-Asn-Thr-Leu-Ile-Ser-Gly-Leu-Gly-Lys-Ala-Gly). A synthetic gene encoding the final cPPR design was optimized for expression in E. coli and synthesized from overlapping oligonucleotides (GeneArt, Life Technologies), as were gene variants encoding cPPRs with altered residues at positions 4 and 34. Protein purification for binding assays Coding sequences for cPPRs were subcloned into pTYB3 and expressed as fusions to an intein and chitin-binding domain in E. coli ER2566 cells (New England Biolabs) [54] . Cells were lysed by sonication in 20 mM Tris-HCl (pH 8.0), 1 M NaCl and 0.1 mM PMSF. Lysates were clarified by centrifugation and incubated for 40 min with chitin beads (New England Biolabs). Beads were washed twice with 20 mM Tris-HCl (pH 8.0), 1 M NaCl, and 0.1 mM PMSF, once with 20 mM Tris-HCl (pH 8.0), 0.5 M NaCl and 0.1 mM PMSF, and once with 20 mM Tris-HCl (pH 8.0), 0.15 M NaCl, and 0.1 mM PMSF. DTT was added to the beads to 50 mM final concentration and the tube was purged with nitrogen gas before incubation at room temperature with gentle rocking for 3 days. Cleaved cPPR protein, free from the intein and chitin-binding domain was collected, transferred into 10 mM HEPES (pH 7.4), 150 mM NaCl, 10% glycerol and further purified by an ÄKTA-Explorer system (GE) using a Superdex 200 10/300 column (GE) with a total bed volume of 120 ml. Pure fractions were pooled and concentrated using Microsep 10 K Omega centrifugal devices (PALL). Protein concentration was determined by the bicichroninic acid (BCA) assay using bovine serum albumin (BSA) as a standard. RNA electrophoretic mobility shift assays Purified cPPR proteins were incubated at room temperature for 30 min with fluorescein labelled RNA oligonucleotides (Dharmacon) in 10 mM HEPES (pH 8.0), 1 mM EDTA, 50 mM KCl, 2 mM DTT, 0.1 mg ml −1 fatty acid-free BSA and 0.02% Tween-20. The following RNA sequences were used: polyA: 5′-(Fl)AAAAAAAAAA-3′; polyC: 5′-(Fl)CCCCCCCCCC-3′; polyG: 5′-(Fl)AAGGGGGGGG-3′; polyU: 5′-(Fl)UUUUUUUUUU-3′; NRE: 5′-(Fl)AUU G UAUAUA-3′; NREG2A: 5′-(Fl)AUU A UAUAUA-3′; NREG2C: 5′-(Fl)AUU C UAUAUA-3′; NREG2U: 5′-(Fl)AUU U UAUAUA-3′; MBNL1: 5′-(Fl)AUGCUUCGCU-3′; MBNL1-CC: 5′-(Fl)AUGC CC CGCU-3′; AAAACAAA: 5′-(Fl) AAAAAA C AAA-3′. Reactions were analysed by 10% PAGE in TAE and fluorescence was detected using a Typhoon FLA 9,500 biomolecular imager (GE). All presented images are representative of results from at least three independent experiments. Protein purification for crystallography Coding sequences for cPPRs were subcloned into pETM30 and expressed as fusions to an N-terminal His tag and glutathione- S -transferase in the E. coli BL21(DE3) strain. The cells were incubated at 18 °C overnight in LB medium following induction with 0.25 mM isopropyl β- D -thiogalactopyranoside. After harvesting by centrifugation at 5,000 g , pellets of induced cells were resuspended on ice in lysis buffer (50 mM sodium phosphate buffer pH 7.5, 1 M sodium chloride, 20 mM imidazole and 5 mM β-mercaptoethanol) supplemented with protease inhibitors (pepstatin 2 μg ml −1 , leupeptin 2 μg ml −1 and phenylmethylsulfonyl fluoride 1 mM), DNase I 10 μg ml −1 and lysozyme 10 μg ml −1 . Cells were lysed using an emulsiflex system (AVESTIN) and cleared by centrifugation at 25,000 g for 30 min at 4 °C. The soluble fraction was purified by affinity chromatography using a 5-ml HisTrap FF crude column (GE Healthcare). Proteins bound to the column were extensively washed with 50 mM sodium phosphate buffer pH 7.5, 300 mM sodium chloride, 20 mM imidazole and 5 mM β-mercaptoethanol. On elution of the protein with washing buffer supplemented with 250 mM imidazole, the fractions were desalted and incubated overnight at 18 °C in presence of TEV protease (1/100 w/w) to cleave the protein tags. The samples were reloaded on a HisTrap FF crude column (GE Healthcare) for removing the tags and the TEV protease. The cleaved cPPR proteins were recovered in the flow-through and concentrated using Amicon 30 kDa MWCO concentrators (Merck Millipore). The concentrated samples were injected on a HiLoad 16/600 Superdex 200 gel-filtration column (GE Healthcare) pre-equilibrated in crystallization buffer (10 mM Tris-HCl pH 7.5, 150 mM NaCl, 5 mM ß-mercaptoethanol). Pure fractions were pooled and concentrated to 5–10 mg ml −1 and either stored in aliquots at −20 °C or used immediately for crystallization trials. Seleno-methionine (SeMet)-labelled cPPR proteins were expressed in the methionine auxotrophic strain B834(DE3) of E. coli using M9 minimal medium with SeMet and then purified as described above. Crystallization and structure determination cPPR protein crystals were obtained using the sitting-drop vapour diffusion technique at 18 °C in 96-well crystallization plates (Swiscii). The drops were prepared by mixing 0.2 μl of the protein solution (at a concentration of 5–15 mg ml −1 ) with an equal volume of crystallization solution and were equilibrated against 35 μl of crystallization solution. cPPR proteins gave diffracting crystals under the following conditions: (1) cPPR-poly(C): 0.1 M MES/imidazole pH 6.1–6.7, 0.03 M CaCl 2 , 0.03 M MgCl 2 , 24–34% PEG4000-glycerol mix (optimized from Molecular Dimensions Morpheus screen, condition 3), (2) (SeMet)-cPPR-NRE: 0.1 M BisTris pH 6.1–6.7, 0.2 M CaCl 2 2·H 2 O, 0–10% pentanediol, 0–16% Formamide (optimized from Hampton Research Index screen, condition 55), (3) cPPR-NRE: 0.1 M BisTris pH 6.1–6.7, 0.2 M CaCl 2 2·H 2 O, 5–30 mM MgSO 4 (optimized from Hampton Research Index screen, condition 55), (4) cPPR-poly(G): 0.1 M BisTris pH 6.1–6.7, 17–22% PEG 3,350 (optimized from Hampton Research Index screen, condition 43) (5) cPPR-poly(A): 0.2 M MgCl 2 , 0.1 M Tris pH 7.0, 10% w/v PEG 8,000 (Molecular Dimensions JCSG- plus screen, condition 20). After optimization, crystals were transferred into cryoprotective buffers before flash freezing in liquid nitrogen. Diffraction data for cPPR protein crystals were collected at the Swiss Light-Source beamline PXIII at 100 K (SLS, Villigen-Paul Scherrer Institute). Crystallographic data are reported in Table 1 . The structure of the SeMet derivative of cPPR-NRE was determined by SAD method using the anomalous signal of the selenium atoms. The data set was indexed, integrated and scaled with the XDS package [55] . Heavy atom location and phasing were performed with the program SHARP [56] . Furthermore, the program SOLOMON [57] was used for phase improvement by solvent flipping. Model building was done using the graphic program COOT [58] . The model was then used for phasing the data sets of cPPR-polyC, cPPR-NRE (high resolution data set) cPPR-polyG and cPPR-polyA protein crystals using the molecular replacement program Phaser from the CCP4 package [59] . The atomic models were refined using the program Phenix [60] . The refinement process included successive rounds of simulated annealing, energy minimization, B-factor and TLS refinements as well as calculation of difference Fourier electron density maps. For (SeMet)-cPPR-NRE and cPPR-NRE protein models, water molecules and ions were added in the late stage of the refinement. The final cPPR protein models show good stereochemistry as indicated by the program PROCHECK with no residue in the disallowed regions of the Ramachandran plot. Thermal shift assay Thermal scanning (25 to 95 °C at 3 °C min −1 ) was performed using a real-time PCR machine (7900HT Fast Real-Time PCR, Applied Biosystems) in 384 well plates and fluorescence intensity was measured after every 15 s. Purified cPPR-NRE and PPR10 were diluted in a buffer containing 10 mM Tris-HCl pH 7.5, 150 mM NaCl and 5 mM MgCl 2 . All assay experiments were made in triplicate in a final volume of 10 μl. Each sample contained 8 μl of buffer, 1 μl of protein solution (10 μg μl −1 for cPPR-NRE and 1 μg μl −1 for PPR10) and 1 μl 100 × SYPRO Orange dye (Invitrogen). PCR plates were sealed and centrifuged before fluorescence intensity measurements. Melting temperatures were calculated using the real-time PCR instrument software provided by Applied Biosystems. How to cite this article: Coquille, S. et al. An artificial PPR scaffold for programmable RNA recognition. Nat. Commun. 5:5729 doi: 10.1038/ncomms6729 (2014). Accession codes . Structure factors and atomic models have been deposited in the Protein Data Bank with the following codes: cPPR-polyA, 4WN4; cPPR-polyC, 4WSL; (SeMet)-cPPR-NRE, 4PJS; cPPR-NRE, 4PJR; cPPR-polyG, 4PJQ.